Trapping and rotating nanoparticles using a plasmonic nano-tweezer with an integrated heat sink Although optical tweezers based on far-fields have proven highly successful for manipulating objects larger than the wavelength of light, they face difficulties at the nanoscale because of the diffraction-limited focused spot size. This has motivated interest in trapping particles with plasmonic nanostructures, as they enable intense fields confined to sub-wavelength dimensions. A fundamental issue with plasmonics, however, is Ohmic loss, which results in the water, in which the trapping is performed, being heated and to thermal convection. Here we demonstrate the trapping and rotation of nanoparticles using a template-stripped plasmonic nanopillar incorporating a heat sink. Our simulations predict an ~100-fold reduction in heating compared with previous designs. We further demonstrate the stable trapping of polystyrene particles, as small as 110 nm in diameter, which can be rotated around the nanopillar actively, by manual rotation of the incident linear polarization, or passively, using circularly polarized illumination. Optical forces have found a wide range of applications in nanoscience. Optical tweezers are widely used for single-molecule force spectroscopy [1] . Optical lattices generated by multibeam interference have been employed for passive particle sorting [2] . Particles have been spun using the angular momentum carried by light [3] , [4] , [5] . However, far-field based optical trapping methods [6] , [7] suffer from the diffraction-limited focused spot size [8] that makes trapping and positioning of nanoscale objects difficult. The trapping potential varies with the cube of the object diameter (for a nanosphere), so small objects require high laser powers. Similarly, positional control with a precision commensurate with object size is difficult, as the potential well in which the object is trapped has a width of roughly half the wavelength [8] . To overcome these problems, the use of the near-fields around photonic and plasmonic structures has been explored [9] , [10] , [11] , [12] , [13] , [14] , [15] . Compared with photonic structures [16] , [17] , [18] , plasmonic devices have the advantages that field enhancement is achieved over a broad range of wavelengths, and using simple free space coupling. The heating associated with plasmon excitation, however, can have substantial effects. Indeed, Garces-Chavez et al . [19] demonstrated trapping using both optical and non-optical (thermophoretic and convective) forces produced by surface plasmon polaritons. Righini et al . [10] trapped beads using surface plasmons on gold pads. The beads were freed from the pads ~1 min after changing the polarization, and it was noted that heating may have a significant role in the trapping process [10] . Ploschner et al . [20] carried out a study of trapping using a plasmonic nanoantenna and suggested that observed localization of particles in (ref. 21 ) may have been due to means other than optical forces. This motivates the development of a plasmonic nanotweezer employing thermal management, as heating limits the maximum optical power that can be used, thereby restricting the magnitude of the optical force or trapping stiffness that can be achieved, and complicates the trapping process. Plasmonic structures are frequently formed on glass substrates, due to their excellent optical properties and low cost. For trapping, however, this leads to two difficulties. Firstly, glass has a comparatively low thermal conductivity ( κ glass ~1 W K −1 m −1 ) [22] , meaning that the illumination intensity must be limited to prevent appreciable water heating. This stops high trapping stiffness from being achieved. As described in the Methods section, we simulate that a water temperature rise of 49 K results from illumination of a gold disk on a glass substrate with a plane wave having an intensity of 1 mW μm −2 . Further details are also given in Supplementary Figure S1 and Supplementary Table S1 . We also observed water boiling and steam bubble generation at a higher illumination intensity, of 8 mW μm −2 , as shown in Supplementary Movie 1 and Supplementary Figure S2 . As we describe later, for the plasmonic nano-tweezer we introduce, there are no thermal effects observed at this illumination level, or even up to ~30 mW μm −2 , the highest intensity we can achieve due to limitations in laser power. Secondly, when transparent substrates are used, significant field enhancement occurs within the substrate, around the bottom corners of the structure. The field distributions are non-optimal, as these are regions that cannot be accessed by the particles to be trapped. Using diamond as the substrate enables the first difficulty to be overcome. Because of its high thermal conductivity ( κ diamond ~1,000 W K −1 m −1 ) [22] , the water temperature rise is predicted to be ~250 times smaller, for the same illumination intensity, with diamond, rather than glass, as the substrate ( Supplementary Table S1 ). However, the second difficulty remains, and another approach is needed. Here we present a design of plasmonic nano-tweezer with an integrated heat sink that overcomes both difficulties discussed above, that is, the heating of water and the non-optimal near-field distribution occurring with previous approaches. We demonstrate a fabrication process, based on template stripping with a reusable master, which yields the nanostructures that comprise the nano-tweezers with high quality and reproducibility. We show experimentally two modes of plasmonic nanoparticle trapping and rotation. In the first, using linearly polarized illumination, we demonstrate the trapping and manual rotation of nanoparticles. In the second, using circularly polarized illumination, we demonstrate that nanoparticles can be trapped and passively rotated, through a conversion from the photon's spin to the particle's orbital momentum. Design The structure we introduce ( Fig. 1a ) comprises a gold nanopillar protruding from a gold film on a copper film formed on a silicon substrate. Gold, copper and silicon have high thermal conductivities ( κ Au =317 W K −1 m −1 , κ Cu =401 W K −1 m −1 , κ Si =148 W K −1 m −1 ) [22] , meaning that the heat generated by plasmon excitation is conducted into the substrate, rather than into the water. Simulations indicate that this heat sinking approach achieves an ~100-fold reduction in water temperature rise, compared with a gold disk on a glass substrate (Methods; Supplementary Fig. S1 and Supplementary Table S1 ). The second difficulty of non-optimal field distribution is also overcome. The dipolar resonance excited by linearly polarized normal-incidence illumination comprises two hot spots at the top edge of the pillar ( Fig. 1b,c ), regions that can be accessed by the particle. 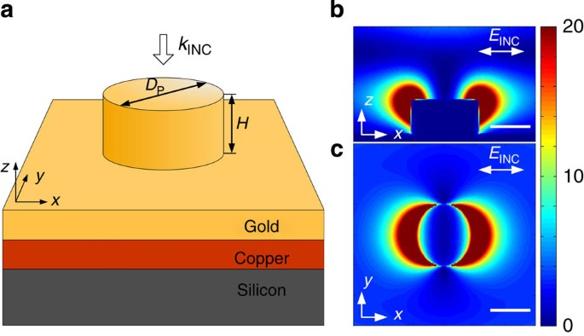Figure 1: Gold nanopillar tweezer. (a) Plasmonic nano-tweezer comprising nanopillar formed on gold film. Underlying copper film and silicon substrate act as heat sink, conducting heat from nanopillar to substrate, thereby minimizing water heating. Nanopillar diameterDPis 280 nm, and heightHis 130 nm. (b,c) FDTD calculation of the electric field intensity distribution resulting from normal incidence plane wave illumination polarized alongx-axis (Einc) atλ=974 nm. Intensity enhancement, that is, intensity normalized to incident intensity |E|2/|EINC|2, is plotted. Peak intensity enhancement is 490 times, although upper limit of colourscale is chosen to be 20 times for visualization. Scale bars, 200 nm. Figure 1: Gold nanopillar tweezer. ( a ) Plasmonic nano-tweezer comprising nanopillar formed on gold film. Underlying copper film and silicon substrate act as heat sink, conducting heat from nanopillar to substrate, thereby minimizing water heating. Nanopillar diameter D P is 280 nm, and height H is 130 nm. ( b , c ) FDTD calculation of the electric field intensity distribution resulting from normal incidence plane wave illumination polarized along x -axis ( E inc ) at λ =974 nm. Intensity enhancement, that is, intensity normalized to incident intensity | E | 2 /| E INC | 2 , is plotted. Peak intensity enhancement is 490 times, although upper limit of colourscale is chosen to be 20 times for visualization. Scale bars, 200 nm. Full size image Fabrication Because the design calls for a gold nanopillar protruding from a gold film, template stripping can be employed in the fabrication process ( Fig. 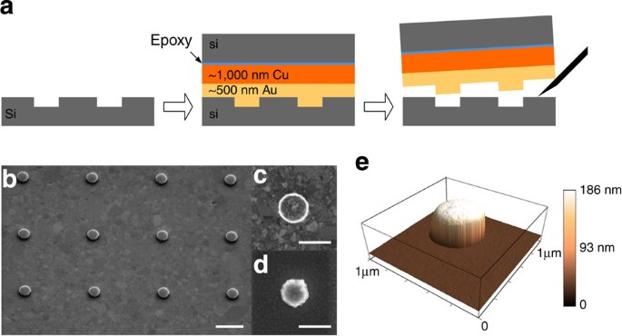Figure 2: Fabrication of gold nano-pillars by template stripping. (a) Fabrication procedure. (b) Scanning electron microscope picture of devices fabricated by template stripping. Scale bar, 1 μm. (c) Zoom in picture of one gold pillar fabricated by template stripping. Scale bar, 300 nm. (d) Scanning electron microscope picture of gold nanopillar fabricated by e-beam lithography and lift-off. Scale bar, 300 nm. (e) atomic force microscope image of template-stripped gold nanopillar. 2a ), with the result shown in Figure 2b . The nanopillars that result ( Fig. 2c ) have more regular shapes and smoother surfaces than nanopillars fabricated by standard lift-off processes ( Fig. 2d ). The quality of the surface morphology is also evident from the atomic force microscope image shown in Figure 2e . A more detailed comparison is shown in Supplementary Figure S3 and Supplementary Table S2 . Figure 2: Fabrication of gold nano-pillars by template stripping. ( a ) Fabrication procedure. ( b ) Scanning electron microscope picture of devices fabricated by template stripping. Scale bar, 1 μm. ( c ) Zoom in picture of one gold pillar fabricated by template stripping. Scale bar, 300 nm. ( d ) Scanning electron microscope picture of gold nanopillar fabricated by e-beam lithography and lift-off. Scale bar, 300 nm. ( e ) atomic force microscope image of template-stripped gold nanopillar. Full size image Trapping and active rotation of nanoparticles In the experiments, the trapping laser beam ( λ =974 nm) is loosely focused onto the gold nanopillars, which are immersed in a colloid solution comprising fluorescent polystyrene spherical nanoparticles. In the experiments in which 110 nm diameter nanoparticles are trapped, the incident laser beam has an average intensity I avg =10 mW μm −2 . 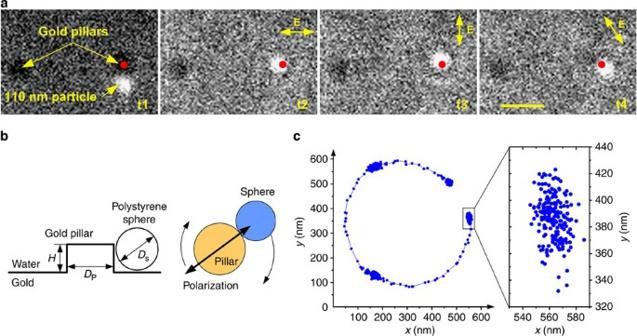Figure 3: Trapping and manual rotation of polystyrene nanospheres by gold nanopillars. (a) Fluorescence images, obtained at successive times, of trapping and rotating 110 nm diameter polystyrene sphere by gold nanopillar. At time t1, sphere is close to nanopillar, but not trapped. At times t2, t3 and t4, sphere is trapped by nanopillar. Input polarization is manually rotated, resulting in sphere rotating clockwise about pillar. Red dots represent position and size of nanopillar. Scale bar, 2 μm. (b) Schematic illustration of trapping and manual rotation of nanosphere by gold nanopillar with linearly polarized illumination.Dp=280 nm andH=130 nm. (c) Left: Centroid of trapped sphere (DS=200 nm) while polarization is being manually rotated. Right: centroid of trapped sphere measured without polarization rotation. Fluorescence images of the trapping process obtained at successive times (t1–t4) are shown as Figure 3a . The sphere appears white, whereas the gold nanopillars appear black. At time t1, the sphere is close to, but is not trapped by, the gold nanopillar, and moves under Brownian motion. At time t2, the sphere has moved sufficiently close to the nanopillar to be drawn into one of the hot spots ( Fig. 1b,c ) by the gradient force and be trapped. The positions of the two hot spots are determined by the polarization of the input laser beam. Here we demonstrate that this can be employed to rotate particles in a precise manner, as shown in Figure 3b . After the sphere is trapped, we manually rotate the input beam polarization during frames t2–t4, resulting in the sphere rotating clockwise around the nanopillar ( Supplementary Movie 2 ). Figure 3: Trapping and manual rotation of polystyrene nanospheres by gold nanopillars. ( a ) Fluorescence images, obtained at successive times, of trapping and rotating 110 nm diameter polystyrene sphere by gold nanopillar. At time t1, sphere is close to nanopillar, but not trapped. At times t2, t3 and t4, sphere is trapped by nanopillar. Input polarization is manually rotated, resulting in sphere rotating clockwise about pillar. Red dots represent position and size of nanopillar. Scale bar, 2 μm. ( b ) Schematic illustration of trapping and manual rotation of nanosphere by gold nanopillar with linearly polarized illumination. D p =280 nm and H =130 nm. ( c ) Left: Centroid of trapped sphere ( D S =200 nm) while polarization is being manually rotated. Right: centroid of trapped sphere measured without polarization rotation. Full size image Analysis of the sphere motion yields information on the trapping process. Because of the small number of fluorophores contained by the 110 nm spheres and the short exposure times needed to capture their motion, the signal-to-noise ratio is not high. We, therefore, instead, performed analysis on trapped 200 nm diameter spheres. Supplementary Movie 3 shows the trapping and rotation of these spheres with an illumination intensity of 5 mW μm −2 . From the movie, the nanosphere centroid position is found as a function of time, and plotted as Figure 3c . It can be seen that the nanosphere makes an approximately circular trajectory about the nanopillar, as the polarization is manually rotated. The trajectory diameter is ~500 nm, which is roughly the sum of the nanosphere ( D s =200 nm) and nanopillar ( D p =280 nm) diameters. This indicates that the nanosphere is trapped by the nanopillar's optical near field and is in direct contact with, or has a very small separation to, the nanopillar. Figure 3c (right side) shows an expanded view of sphere position measured when the polarization is not being rotated. It can be seen that the sphere is more tightly confined in the radial direction (var( x )=14 nm 2 ) than in the tangential direction (var( y )=68 nm 2 ). This is because the field gradient is stronger along the radial direction than the tangential, as shown in Figure 1c . Because the camera is not operating fast enough to capture the instantaneous positions of the moving particle, these measured variances are reduced by the motion blur during a long exposure time (30 ms). If we approximate the trapping potential as parabolic and assume that Stokes' drag applies, the trapping stiffness can be extracted from these measurements using the method introduced by Wong and Halvorsen [23] that corrects for motion blur. This yields trapping stiffnesses in the radial and tangential directions of k r =11 pN μm −1 and k t =3 pN μm −1 . These represent a lower bound of trapping stiffness, however, as the Stokes' drag assumption, that is, that the nanosphere's drag coefficient is 6 πηα =1.88×10 −9 (N s m −1 ), where η is the dynamic viscosity of water and α is the radius of the nanosphere, is strictly correct only for a sphere surrounded by a homogeneous medium. Near a planar surface, Faxén's law predicts that the drag coefficient increases with a fifth order polynomial dependence on the inverse of the particle–surface separation [1] . This distance varies with time owing to Brownian motion, but assuming an average gap of 4 nm, the drag coefficient increases by a factor of 2.7 and the corrected trapping stiffnesses are k r =19 pN μm −1 and k t =4.8 pN μm −1 . For curved surfaces, the drag coefficient increases even more, so these numbers still represent a lower limit on the true stiffness. Illumination of the nanopillar by linear polarization generates two hot spots on opposite sides of the pillar. We demonstrate that this enables the simultaneous trapping of two spheres, as shown in Supplementary Movie 4 . The centre-to-centre distance between them is ~480 nm. Because of the limited resolution of the microscope, two spheres merge to appear as an ellipse. It can be seen, however, that the ellipse rotates as the polarization is manually rotated, confirming that the two spheres rotate together. In the experiments, an array period of 5 μm is used. Very similar performance might be expected, though, with a nanopillar array with a period of 1 μm, for trapping of two particles per nanopillar. For an illumination intensity of 5 mW μm −2 , the power associated with each trapping site would be 2.5 mW. From the estimated trapping stiffnesses in previous experiment: k r =19 pN μm −1 and k t =4.8 pN μm −1 , the normalized trapping stiffnesses would be 7.6 and 1.9 pN μm −1 mW −1 in radial and tangential directions, which are more than an order of magnitude higher than conventional optical tweezers [24] . Passive rotation of nanoparticles Using circularly polarized illumination, nanosphere rotation in a passive manner becomes possible. Unlike the active rotation method described above, manual polarization rotation is unnecessary. The two hot spots rotate at the laser frequency, meaning that the time averaged electric field intensity comprises a hot spot ring ( Fig. 4a ). This leads to a constant energy flow clockwise or anti-clockwise, depending on the handedness of the incident circular polarization. 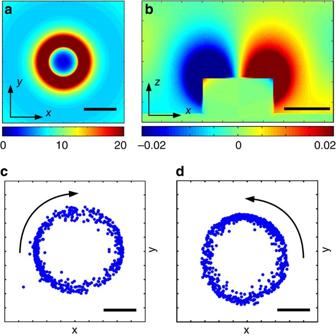Figure 4: Passive rotation of polystyrene spheres by gold nanopillar. (a) FDTD calculation of electrical field intensity enhancement|E|2/|EINC|2distribution resulting from circularly polarized illumination atλ=974 nm. (b) FDTD calculation ofy-component of Poynting vector around nanopillar with left circularly polarized illumination. Colourbar is in units of W m−2, and take the incident illumination to have an electric field with amplitude |E|=1 V m−1. (c,d) Centroid tracking inx–yplane of 340 nm sphere trapped and rotated by nanopillar with right and left circularly polarized illumination, respectively.H=130 nm,DP=280 nm,DS=340 nm,Iavg=5 mW μm−2. Arrows indicate the rotation directions. Scale bars, 200 nm. In Figure 4b , the y -component of the Poynting vector is shown for left circularly polarized illumination of the nanopillar. It can be seen that there is an anti-clockwise energy flow around the nanopillar. It should be expected, therefore, that trapped particles will be driven by the scattering force to rotate in the same direction as the energy flow. Figure 4: Passive rotation of polystyrene spheres by gold nanopillar. ( a ) FDTD calculation of electrical field intensity enhancement| E | 2 /| E INC | 2 distribution resulting from circularly polarized illumination at λ =974 nm. ( b ) FDTD calculation of y -component of Poynting vector around nanopillar with left circularly polarized illumination. Colourbar is in units of W m −2 , and take the incident illumination to have an electric field with amplitude | E |=1 V m −1 . ( c , d ) Centroid tracking in x–y plane of 340 nm sphere trapped and rotated by nanopillar with right and left circularly polarized illumination, respectively. H =130 nm, D P =280 nm, D S =340 nm, I avg =5 mW μm −2 . Arrows indicate the rotation directions. Scale bars, 200 nm. Full size image We demonstrate this experimentally. Supplementary Movies 5 and 6 , and Supplementary Figure S4 show experimental results in which a 340-nm diameter polystyrene particle is trapped and rotated clockwise and anti-clockwise using right and left circularly polarized illumination, respectively. An illumination intensity of 5 mW μm −2 is used. Histograms of particle centroid position ( Fig. 4c,d ) from these movies show that they follow circular trajectories. However, it can be seen that the particle positions are not uniformly distributed around the circle, because the field is not perfectly uniform around the nanopillar. Non-uniformity of the field modifies both the gradient and scattering forces, preventing smooth rotation. Because Brownian motion also acts on the particle, the rotation happens in a burst manner randomly. Over the measurement period of 30 s, the average speed of anticlockwise rotation and clockwise rotation as shown in Figure 4c,d are 4.3 and 5.7 revolutions per second, respectively. The optical torque exerted on a trapped particle is given by τ = r × F = r ×( μv ), where r =310 nm is the radius of the rotation track, F is the tangential force, μ= 6 πηα is the drag coefficient and v is the average velocity. From the experimental results, we find the optical torque on a 340 nm polystyrene sphere is 9.7 pN nm, for an illumination intensity of 5 mW μm −2 . Using finite-difference time-domain (FDTD) simulations and the Maxwell stress tensor method, the expected optical torque with this structure is found to be 80 pN nm, as shown in Supplementary Figure S5 . The experimental results are therefore 8 times smaller than the theoretical prediction. Two possible reasons could be responsible for this discrepancy: first, the drag coefficient being underestimated, as mentioned earlier; second, one would expect the non-uniform field intensity around the nanopillar to lead to an extra gradient force that prevents fast rotation. In summary, we demonstrate the trapping of spheres with diameters as small as 110 nm using a template stripped plasmonic nanopillar that produces dramatically less water heating than previous designs. The materials (gold, copper and silicon) under the nanopillar have high thermal conductivities, enabling heat to be conducted from it in an effective manner. We demonstrate that the trapped particles can be actively rotated around the nanopillar by manually rotating the linear polarization of the input beam, opening a new way of controlling the position of a trapped particle. On the other hand, using circularly polarized illumination, trapped particles can be rotated passively, that is, without the need for manual intervention. The nanopillar, therefore, presents a means of converting the angular momentum of the input illumination to the orbital momentum of a nanoparticle, thereby introducing a nanoscale motor functionality. Additionally, the simultaneous two particles trapping by two hot spots on a single gold nanopillar demonstrated the trapping of two particles with a distance smaller than the diffraction-limit, which makes super-resolution optical trapping possible. We anticipate that the trapping of particles with diameters well below 100 nm is possible, as smaller particles should interact even more efficiently with the near-field hot spots. In addition, the heat sink makes the use of higher optical powers possible. However, if we want to extract quantitative information from such an experiment, the practical difficulty lies in the motion detection of smaller particles, and a more sensitive camera or a different detection scheme (for example, based on a quadrant photodetector) will be required. A number of interesting possibilities exist for extending this work. Elongated, rather than circular, nanopillars with two resonance frequencies could enable wavelength multiplexing of the trapping. Pairs of nanopillars separated by small gaps [25] could permit very high field enhancements to be achieved for trapping small particles. Lastly, using arrays of nanopillars, the simultaneous trapping of a large number of nanoparticles could be carried out. If the spacing between nanopillars is chosen appropriately, the arrays also present the opportunity for larger field enhancement [26] , [27] , and therefore stronger optical forces, than single isolated nanopillars. Numerical simulation of thermal effects The Ohmic loss in plasmonic devices is an important issue because it can lead to two side effects that prevent stable trapping: thermal convection and overheating of water. To understand, and therefore minimize, the heating accompanying plasmon excitation, we model it numerically. The geometry is shown in Supplementary Figure S6a . A circular-shaped gold disk sits on a substrate in the centre of a water-filled chamber. Because the geometry is axially symmetric, the three-dimensional model of Supplementary Figure S6a can be simplified to a two-dimensional model, as shown in Supplementary Figure S6b . Because of the small chamber dimension (~1 mm) and the slow convection flow velocity (~10 μm s −1 ), the Reynolds number in this system is very small (~0.01). A stable convection velocity field can therefore be solved by finding steady-state solutions of the Navier–Stokes equations [28] . Using the Boussinesq approximation, it can be further simplified to be the problem of incompressible flow with the extra volume force induced by buoyancy [28] . Combining this with the conduction–convection equation for heat transfer [28] , the temperature distribution and convection velocity field can be readily solved numerically using the fluid dynamics module provided by Comsol Multiphysics. In the numerical calculation, the outer boundaries are set at to be at room temperature and the gold pillar is the only source of heat. The absorbed power, which is converted to heat, is calculated by P = C abs × I , where C abs is the absorption cross-section obtained from FDTD simulations and I is the illumination intensity. We make the assumption that the heating power is uniformly distributed throughout the volume of the gold nanopillar, which is reasonable because of the high thermal conductivity of gold. The simulation results are shown in Supplementary Figures S1, S7, S8 and summarized in Supplementary Table S1 . Device fabrication The fabrication procedure is shown in Figure 2a : The silicon template is first fabricated by e-beam lithography and reactive ion etching. Native oxide on the surface then results from the sample being exposed to the ambient environment. Gold (500 nm) and copper (1,000 nm) are then deposited by e-beam evaporation. A piece of single crystal silicon is then stuck on to the copper film with a very thin layer of epoxy (EPO-TEK 330, Epoxy Tech). Finally, the whole structure is stripped from the template using a blade. Experimental setup In the experimental setup (as shown in Supplementary Fig. S9 ), a laser beam ( λ =974 nm) is focused by a microscope objective (Nikon, NA=0.45, ×50) onto the gold nanopillar. The laser beam does not fill the objective back aperture, resulting in the focused spot having a 1/e 2 intensity diameter of ~3 μm, which relaxes the alignment tolerance. The chamber between substrate and glass cover slide is filled with a diluted colloid solution (carboxylate-modified microspheres, Invitrogen) to which surfactant (0.5% by weight, Triton X100, Sigma-Aldrich) and 5 mM NaCl are added to prevent adhesion and screen surface charges, respectively. A second laser beam ( λ =532 nm) is loosely focused by the objective on the sample to excite fluorescence from the colloidal particles, which is imaged onto a CCD camera (PhotonMax, Princeton Instruments). The set-up enables the positions of particles to be determined with high precision. Numerical calculation of optical torque The numerical calculation of optical force is conducted in the following way: First, the electric and magnetic fields are calculated around a sphere in the vicinity of the gold nanopillar by FDTD simulations (Lumerical FDTD). Second, the force on the sphere is found by the Maxwell stress tensor from the fields. The FDTD simulation geometry is shown in Supplementary Figure S10 . The simulations indicate that the optical forces attract the sphere down towards the surface. The gap between sphere and bottom surface is chosen to be 4 nm. The field distributions, E Ex and E Ey , resulting from x - and y -polarized plane wave illumination are found by separate FDTD simulations, as shown in Supplementary Figure S10b,c . The optical field under left and right circular polarization excitation can then be found as: E left = E Ex + j * E Ey , E right = E Ex − j * E Ey , as shown in Supplementary Figure S11 . Using the Maxwell stress tensor method, the optical force can be obtained, as shown in Supplementary Figure S12 . To facilitate comparison, the simulation parameters are chosen to be those used in the experiments on the passive rotation of 340 nm polystyrene particles. The optical torque on the sphere can be calculated from τ = r × F y , where r =310 nm+gap is the radius of the rotation track, as shown in Supplementary Figure S5 . How to cite this article: Wang, K. et al . Trapping and rotating nanoparticles using a plasmonic nano-tweezer with an integrated heat sink. Nat. Commun. 2:469 doi: 10.1038/ncomms1480 (2011).